Mechanical gate control for atom-by-atom cluster assembly with scanning probe microscopy Nanoclusters supported on substrates are of great importance in physics and chemistry as well as in technical applications, such as single-electron transistors and nanocatalysts. The properties of nanoclusters differ significantly from those of either the constituent atoms or the bulk solid, and are highly sensitive to size and chemical composition. Here we propose a novel atom gating technique to assemble various atom clusters composed of a defined number of atoms at room temperature. The present gating operation is based on the transfer of single diffusing atoms among nanospaces governed by gates, which can be opened in response to the chemical interaction force with a scanning probe microscope tip. This method provides an alternative way to create pre-designed atom clusters with different chemical compositions and to evaluate their chemical stabilities, thus enabling investigation into the influence that a single dopant atom incorporated into the host clusters has on a given cluster stability. Nanoclusters supported on substrates are of great importance in physics and chemistry as well as in technical applications, such as single-electron transistors [1] , [2] , nanocatalysts [3] , [4] , [5] and quantum computing devices [6] . The properties of nanoclusters are highly sensitive to size and chemical composition. Despite their inert bulk properties, for example, nanosized Au clusters exhibit high catalytic activities for a wide variety of chemical reactions [3] , showing clear quantum size effects on catalytic behaviour [5] . The development of methods to fabricate atomically well-defined clusters is therefore necessary for a fundamental understanding of their properties and for designing better materials and devices. Various approaches have been developed to create nanoclusters with different functionalities on surfaces. Among these methods, the self-assembling is the most widely used method for fabricating nanoclusters, where atoms/molecules are evaporated onto a surface followed by thermal annealing, leading to the spontaneous formation of clusters [7] . To unveil the unique properties of these clusters in practical applications, it is essential to control their size and uniformity. Although the uniformity of cluster arrays has been achieved using the so-called template-induced cluster formation method [8] , [9] , these methods do not provide direct access to the precise determination of the number of atoms involved in a cluster structure once they are deposited on surfaces. Complementary to these methods, the scanning probe method offers precise positioning capabilities with atomic precision [10] . These capabilities have led to the creation of various artificial nanostructures atom-by-atom, mainly at cryogenic temperatures [11] , [12] , [13] , [14] . This method was later extended to room temperature (RT) by means of atomic force microscopy (AFM) [15] , which provides an opportunity to directly measure the forces that induce the atomic motion in the manipulation process [16] , [17] , [18] . Despite these achievements, assembly of the well-defined clusters exhibiting high thermal stability at RT and the precise determination of the cluster size and hence of the number of atoms involved in a cluster structure remains a challenging task [19] . More importantly, assembling of atomically well-defined clusters from multi-elements at RT has not been demonstrated yet despite their wide range of technical applications. The investigation of the structure and the stability of these bimetallic clusters can contribute to our understanding of the interaction of the doped atom with the metal clusters. In this study, we propose an alternative approach to the assembly of various nanoclusters atom-by-atom using the tip of a scanning probe microscope (SPM) at RT. This method is based on the transfer of single diffusing atoms among nanospaces (NSs) governed by gates, which can be opened in response to the chemical interaction force with the SPM tip. This method provides a way to create pre-designed atom clusters with different chemical compositions and to evaluate their chemical stabilities. Transfer of diffusing adsorbates by atom gating Half-unit cells (HUCs) of the Si(111)-(7 × 7) surface serve as NS arrays to confine individual adsorbates diffusing on the surface. Single atoms deposited on the surface, such as group IV elements (Si, Sn and Pb) and noble metals (Ag and Au), thermally diffuse within the NSs at RT as demonstrated in Fig. 1 . A potential energy barrier existing between NSs prohibits inter-NS thermal diffusion. The diffusion rate within the NS is so large that a SPM cannot resolve the specific adsorption sites offered by the surface at RT [20] (further information can be found in Supplementary Note 1 ). The different adsorbate atoms on the surface appear differently in the SPM images owing to differences in their diffusion properties ( Fig. 1b–i ). 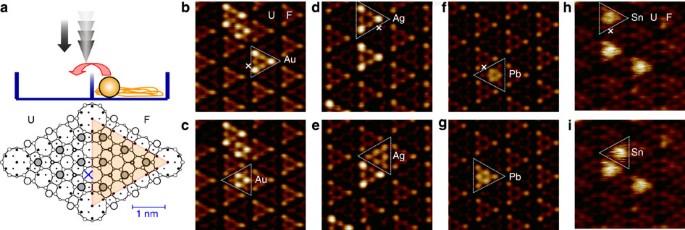Figure 1: Demonstrations of the transfer of a single atom by gate control. (a) A HUC in the Si(111)-(7 × 7) surface works as a NS of an equilateral triangle with side lengths of 2.7 nm. F and U denote faulted and unfaulted HUC, respectively. The adsorbate atom travels among the various potential minima in a NS; these minima are known to be multi-coordinate sites rather than the tops of Si adatoms and rest atom sites26. The tip gradually approaches the position as indicated by a cross in the Si(111)-(7 × 7) unit cell for the gate-opening process. This process initiates the atom transfer between two NSs. (b–g) The corresponding STM images atVs=−1,000 mV exemplify the atom transfer ability using gate control for (b,c) Au, (d,e) Ag and (f,g) Pb. The tunnelling current set points are (b,c) 30, (d,e) 50 and (f,g) 40 pA. The white dashed triangles mark the initial (b,dandf) and final (c,eandg) locations of adsorbates transferred by gate control. (h,i) AFM images showing Sn atom transfer by atom gating with AFM tip atVs=0 V. The acquisition parameters weref0=153,972.5 Hz,k=25.2 N m−1,A=198 Å and Δf=−2.1 Hz. Figure 1: Demonstrations of the transfer of a single atom by gate control. ( a ) A HUC in the Si(111)-(7 × 7) surface works as a NS of an equilateral triangle with side lengths of 2.7 nm. F and U denote faulted and unfaulted HUC, respectively. The adsorbate atom travels among the various potential minima in a NS; these minima are known to be multi-coordinate sites rather than the tops of Si adatoms and rest atom sites [26] . The tip gradually approaches the position as indicated by a cross in the Si(111)-(7 × 7) unit cell for the gate-opening process. This process initiates the atom transfer between two NSs. ( b – g ) The corresponding STM images at V s =−1,000 mV exemplify the atom transfer ability using gate control for ( b , c ) Au, ( d , e ) Ag and ( f , g ) Pb. The tunnelling current set points are ( b , c ) 30, ( d , e ) 50 and ( f , g ) 40 pA. The white dashed triangles mark the initial ( b , d and f ) and final ( c , e and g ) locations of adsorbates transferred by gate control. ( h , i ) AFM images showing Sn atom transfer by atom gating with AFM tip at V s =0 V. The acquisition parameters were f 0 =153,972.5 Hz, k =25.2 N m −1 , A =198 Å and Δ f =−2.1 Hz. Full size image The clusters with predetermined compositions, such as Au 12 , Ag 12 and Au 5 Pb, can be formed by collecting single atoms from the surrounding NSs into a predefined NS with successive gate controls. Hereafter, Au N represents the Au cluster with N Au atoms and the term ‘cluster’ refers to an ensemble of foreign atoms bonded to the Si(111)-(7 × 7) surface. An adsorbate diffusing within a NS can be transferred to an adjacent NS by the tip proximity near the border, but slightly shifted away from the NS where the diffusing atom is located. The gate associated with the potential energy barrier that hinders the mobility of an adsorbate between NSs can be opened by the following consecutive steps. First, the tip is positioned over the predefined site marked with a cross as in Fig. 1a , and then the tip-to-surface distance is gradually decreased. In each gating attempt, this process is repeated until the diffusing atom is successfully transferred into the desired NS. The scanning tunnelling microscopy (STM) images in Fig. 1b,c exemplify the gating process for a Au atom diffusing in a NS (marked by a white dashed triangle). Figure 1b displays three Au atoms. Two of them are located in the faulted HUCs and one in the unfaulted HUC. Three HUCs with Au atoms appear brighter than the bare HUCs. This is attributable to the topographic as well as the electronic structure modifications induced by Au atoms that are diffusing much faster than the scanning speed of the SPM tip, similar to what was observed in a previous study [21] . Atom gating performed over the position marked by the cross in Fig. 1b results in a transfer of a Au atom to an adjacent NS without any surface or tip structural modifications (see Fig. 1c ). We achieved such atom transfers by atom gating for other elements, such as Ag, Pb, Sn and Si atoms (see Fig. 1d,e for Ag and Fig. 1f,g for Pb; also see Supplementary Fig. 1 , Supplementary Note 2 , Supplementary Movies 1 and 2 ). Although we have used only five different elements to demonstrate the gating process on the Si(111)-(7 × 7) surface at RT, this method can be applied, in principle, to other groups of elements. The main requirement that is needed for a successful gating process is the confinement of the adsorbates within a HUC without totally suppressing their mobility inside the HUCs. Figure 1h,i shows AFM images demonstrating the ability to position a single Sn atom using atom gating without a tunnelling current ( I t ) under 0 V bias. The Sn atom can be successfully relocated into the predetermined NS using an AFM tip. This is a strong evidence that the gating operation is not caused by I t . Distance spectroscopy during atom gating The dynamical evolution of the atomic process involved in atom gating can be obtained from the distance dependence of I t ( I t ( z )). 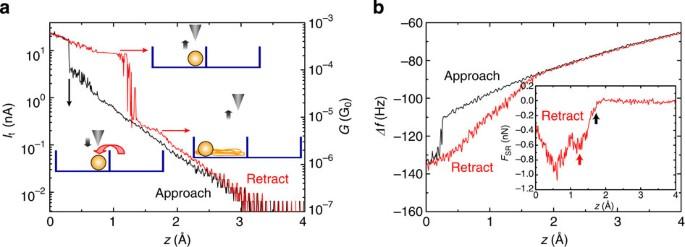Figure 2: STM and AFM observables during atom gating. (a) TypicalIt(z) curves acquired with static STM atVs=−500 mV, revealing the evolution of the current (left axis) and conductance (right axis) during the Au atom gating process with the STM tip as a function of the tip–sample relative displacement. HereG0=2e2/h=(12,906 Ω)−1. The spectroscopic measurements were performed over the site near the boundary of NSs, but slightly shifted away from the NS occupied by a Au atom. The inset schematics inashow the Au atom dynamics during the approach and retraction cycle of the tip (Au atom jump, Au atom trap and release). (b) The variation of the Δfsignal as a function of the tip–sample distance during approach and retraction acquired with AFM. The inset inbshows the short-range force extracted from the Δf(z) curve, revealing the characteristic forces attributed to the trapping of a Au atom (black arrow) and junction formation by the chemical bond between the tip and the Au atom (red arrow). To extract the short-range force, the long-range background part, which is estimated from the approach Δf(z) curve on the bare Si surface, was subtracted from the retraction Δf(z) curve. It was then converted to the short-range force37. We define the origin ofzas the closest distance in data acquisition (no physical meaning). The acquisition parameters weref0=144,412.4 Hz,k=19.8 N m−1,A=114 Å andVs=−500 mV. Figure 2a illustrates the representative semi-logarithmic I t ( z ) curves recorded during the gating of Au by STM, which is acquired over the position marked by a cross in Fig. 1b . The I t ( z ) curve follows the characteristic exponential increase with distance as the tip approaches above the bare Si surface (black curve). The most striking feature in Fig. 2a is the discontinuous jump observed at z =0.3 Å. We ascribed the observed jump to the Au atom hopping from the initial NS to the adjacent empty NS below the tip; this can be explained as follows. Before the gate-opening process, the diffusing Au atom frequently visits adsorption sites close to the boundary between two NSs. When the gate is opened in response to the tip interaction at close proximity to the surface, the Au atom in the instant of closest approach to the boundary can hop to the adjacent NS. The Au atom is then locally trapped under the STM tip by a chemical bonding force. Thereby an atomic junction of the tip–Au–Si surface is formed. The formation of this atomic junction gives rise to a sudden increase in I t , as encountered in our experiments. As the tip–surface separation further decreases ( z <0.3 Å), I t increases with a smaller slope, which signifies that the tunnelling barrier collapses and ballistic current starts to flow through the junction. Figure 2: STM and AFM observables during atom gating. ( a ) Typical I t ( z ) curves acquired with static STM at V s =−500 mV, revealing the evolution of the current (left axis) and conductance (right axis) during the Au atom gating process with the STM tip as a function of the tip–sample relative displacement. Here G 0 =2 e 2 / h =(12,906 Ω) −1 . The spectroscopic measurements were performed over the site near the boundary of NSs, but slightly shifted away from the NS occupied by a Au atom. The inset schematics in a show the Au atom dynamics during the approach and retraction cycle of the tip (Au atom jump, Au atom trap and release). ( b ) The variation of the Δ f signal as a function of the tip–sample distance during approach and retraction acquired with AFM. The inset in b shows the short-range force extracted from the Δ f ( z ) curve, revealing the characteristic forces attributed to the trapping of a Au atom (black arrow) and junction formation by the chemical bond between the tip and the Au atom (red arrow). To extract the short-range force, the long-range background part, which is estimated from the approach Δ f ( z ) curve on the bare Si surface, was subtracted from the retraction Δ f ( z ) curve. It was then converted to the short-range force [37] . We define the origin of z as the closest distance in data acquisition (no physical meaning). The acquisition parameters were f 0 =144,412.4 Hz, k =19.8 N m −1 , A =114 Å and V s =−500 mV. Full size image During the tip retraction (red curve), I t ( z ) follows the approach curve in the range of z <0.3 Å, and continues to decrease with a smaller slope beyond the distance where the Au atom hopped. A plateau region is observed around z =1 Å, where the Au atom is still trapped and the atomic junction is preserved. This atomic junction is stabilized by the chemical bonding force, which is evident in the relatively low noise level in the plateau region (further discussion can be found in Supplementary Note 3 ). We obtained G =2.2 × 10 −4 G 0 as the quantized conductance through a single Au atomic junction, which is much smaller than the one obtained in pure gold atomic junctions where the conductance is close to 1 G 0 (ref. 22 ). The observed small conductance was attributed to the energy level mismatch between the Au and Si surfaces (further discussion can be found in Supplementary Note 4 ). As the tip is retracted further from the plateau region, the I t ( z ) curve fluctuated around z =1.2 Å. The fluctuations suggest the presence of a stochastic trap and release of the Au atom in the junction by the tip. Beyond this transition region, the chemical bond arising between the Au atom and the tip is completely broken, and the Au atom thermally diffuses within the NS all of the time. Consequently, the I t value drops by one order of magnitude. Hereafter, I t decreases as the tip-to-surface distance increases following the basic tunnelling law. The characteristic features observed in the I t ( z ) curves are remarkably identical for different elements used for cluster assembling, thus pointing towards a common mechanism for atom gating. To further elucidate the triggering mechanism of the gating and to quantify the force required to trap the diffusing Au atom under the tip, we performed force spectroscopic measurements using AFM/STM. We simultaneously recorded frequency shift (Δ f ), current and energy dissipation during a gating operation ( Fig. 2b and Supplementary Fig. 2 ). When the oscillating tip approaches the surface for atom gating, all recorded signals jump at around z =0.3 Å, which is the signature of a Au atom hopping from a neighbouring NS. It should be pointed out that once the Au atom is transferred to the NS below the tip, the tip traps and releases the Au atom in each tip oscillation cycle owing to the large cantilever oscillation amplitude used in our experiment (see Supplementary Note 5 and Supplementary Movie 3 ). We determined the threshold force required to trap a single diffusing Au atom below the tip as F SR =−0.1 nN. This was obtained from the short-range force during tip retraction at the distance above which the trapped Au atom diffuses freely within the NS without any further trapping by the tip (see the black arrow in the inset of Fig. 2b , Supplementary Fig. 2 and Supplementary Note 5 ). Moreover, the interaction force stabilizing the atomic junction between the tip and the Au atom can be estimated to be F SR =−0.6 nN (marked by the red arrow), which is in the class of a chemical bonding force [23] . At closer distances, the second force minimum appears in F SR ( z ) curve, which can be attributed to relaxations of the tip apex (see Supplementary Fig. 2 and Supplementary Note 5 ). From the measured force magnitude and the ability to transfer single adsorbates without tunnelling current (see Fig. 1h,i ), we conclude that the gating mechanism is a purely mechanical effect. Here the term ‘mechanical effect’ indicates that the tunnelling current and the electric field do not play any role in the atom gating process. The formation of the chemical bond between the outermost apex atom and the adsorbate atom on the surface weakens the adsorbate bonds with the underlying Si atoms [16] , leading to a local reduction of the energy barrier so that thermal energy enables atom hopping across the gate. Assembly of clusters composed of a defined number of atoms We can fabricate complex atom clusters by the gating technique as described above. Movies showing the assembly of these clusters are available in Supplementary Movies 4–9 . An example, the assembly of Au N clusters ( N =1–12) with most stable forms, is demonstrated in Fig. 3a . These clusters were assembled by bringing N Au atoms into the predetermined NS one-by-one by successive gate operations (see Supplementary Note 6 ). Atom-by-atom assembly allows us to study the dependence of the cluster stability on the size of clusters or the number of atoms that compose them. While Au 1 –Au 3 shows quick thermal diffusion, Au 4 and Au 7 –Au 12 remain stable structures and no changes were observed in their appearance within several hours. On the other hand, Au 5 and Au 6 are relatively stable within the scanning time scale, but in several minutes, conformational changes in the structures of the clusters into the equivalent forms take place by following the mirror and threefold symmetry of the Si(111)-(7 × 7) surface. This type of transformation takes place by collective diffusion of the cluster atoms. 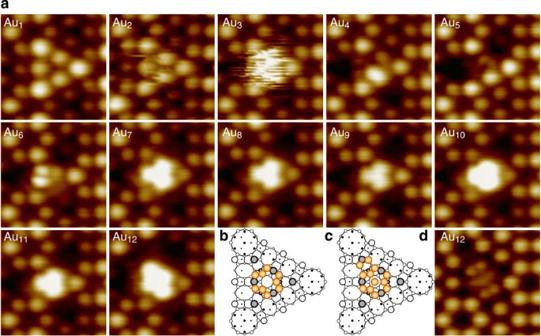Figure 3: Assembly of Au atom clusters by the successive atom gating. (a) STM filled-state images of typical Au1–Au12clusters assembled by gate control (acquired atVs=−500 mV andIt=30 pA). (b) Schematic representation of the structure model for Au9effectuated by Ghoseet al.27In this model, six Au atoms are located inside the basin (close to the H3 site) and the other three reside over the symmetry axes by bonding to the other Au atoms. Au atoms do not participate in bond formation with corner adatoms. (c) Schematic representation of a possible structure model for Au12. (d) STM empty-state image of Au12cluster atVs=1,000 mV andIt=40 pA. Figure 3: Assembly of Au atom clusters by the successive atom gating. ( a ) STM filled-state images of typical Au 1 –Au 12 clusters assembled by gate control (acquired at V s =−500 mV and I t =30 pA). ( b ) Schematic representation of the structure model for Au 9 effectuated by Ghose et al. [27] In this model, six Au atoms are located inside the basin (close to the H3 site) and the other three reside over the symmetry axes by bonding to the other Au atoms. Au atoms do not participate in bond formation with corner adatoms. ( c ) Schematic representation of a possible structure model for Au 12 . ( d ) STM empty-state image of Au 12 cluster at V s =1,000 mV and I t =40 pA. Full size image Au 7 –Au 11 atom clusters look identical to each other, with threefold symmetry in the filled-state STM images, and they resemble the self-assembled Au clusters previously observed in refs 24 , 25 . In that study [25] , the structure model was determined based on the first-principle calculations and the number of Au atoms in the clusters was estimated as six, which is not consistent with our results. Previous investigations showed that metallic elements such as Au and Ag interact with multiple Si atoms to saturate the maximum number of dangling bonds by adsorbing at high coordination sites [26] . A favourable structure model for Au 9 cluster was previously proposed (also depicted in Fig. 3b ) on the basis of X-ray diffraction experiments [27] . The lack of their participation in chemical bonding with corner adatoms and their three-lobe appearance in our STM images suggest that this structure model can serve as a possible basis for structure models for Au 7 –Au 11 . In contrast, the apparent threefold symmetry is broken for Au 12 since one of the corner adatoms starts to participate in bond formation. The Au 12 structure still has a mirror symmetry in both filled- and empty-state STM images (see Fig. 3d ). On the basis of this information and the proposed model for Au 9 cluster [27] , we propose a structure model for Au 12 cluster. The two Au atoms are placed near a corner Si adatom site, and are located symmetrically with respect to the mirror plane. The additional one Au atom is placed at the centre of the HUC. The resulting structure model shown in Fig. 3c fulfils a mirror symmetry as observed by the STM. The precise control of single Au atoms as demonstrated here enables us to determine the exact number of atoms forming each cluster, thus providing accurate information for future calculations to construct possible structure models. Although we did not determine the capacity of a HUC that can accommodate maximum number of Au atoms, we could assemble Au clusters containing up to 17 Au atoms (see Fig. 4e–k ). 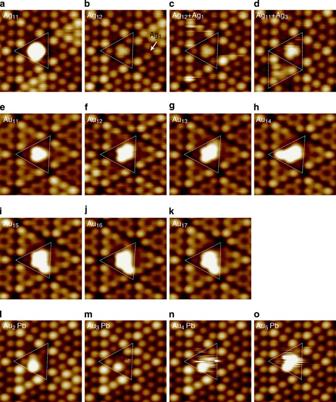Figure 4: The dependence of the cluster stability on composition. (a–d) Series of STM images showing the influence of Ag atom transfer into a NS nearby to the existing Ag cluster formed at the unfaulted HUC of Si(111)-(7 × 7). (a) Ag11; (b) transfer of one Ag atom into an adjacent NS leads to the formation of Ag12; (c) transfer of an additional Ag atom into a neighbouring NS occupied by Ag12does not allow Ag13cluster formation; (d) addition of two Ag atoms into the neighbouring NS occupied by Ag12creates two cluster arrays of Ag11and Ag3. (e–k) STM images showing the Au11–Au17clusters assembled at the unfaulted HUC. (l–o) STM images of multi-element atom clusters showing the influence of a single Pb atom on the stability of Au2–Au5clusters assembled by atom gating control. The acquisition parameters were (a–d)Vs=−1,000 mV andIt=50 pA; (e–k)Vs=−1,000 mV andIt=30 pA; (l–o)Vs=−1,000 mV andIt=30 pA. Figure 4: The dependence of the cluster stability on composition. ( a – d ) Series of STM images showing the influence of Ag atom transfer into a NS nearby to the existing Ag cluster formed at the unfaulted HUC of Si(111)-(7 × 7). ( a ) Ag 11 ; ( b ) transfer of one Ag atom into an adjacent NS leads to the formation of Ag 12 ; ( c ) transfer of an additional Ag atom into a neighbouring NS occupied by Ag 12 does not allow Ag 13 cluster formation; ( d ) addition of two Ag atoms into the neighbouring NS occupied by Ag 12 creates two cluster arrays of Ag 11 and Ag 3 . ( e – k ) STM images showing the Au 11 –Au 17 clusters assembled at the unfaulted HUC. ( l – o ) STM images of multi-element atom clusters showing the influence of a single Pb atom on the stability of Au 2 –Au 5 clusters assembled by atom gating control. The acquisition parameters were ( a – d ) V s =−1,000 mV and I t =50 pA; ( e – k ) V s =−1,000 mV and I t =30 pA; ( l – o ) V s =−1,000 mV and I t =30 pA. Full size image The cluster structures and their stabilities are strongly dependent on the elements that constitute the clusters. Figure 4a–d and Fig. 4e–k compare the stability of distinct types of clusters formed by the individual Ag and Au atoms, respectively. The assembly sequences of these clusters can be found in Supplementary Notes 6 and 7 . Ag 12 formed by atom gating is shown in Fig. 4b . A threefold symmetry in the structure of the Ag 12 cluster is observed, which is clearly different from Au 12 ( Fig. 4f ), although both Ag and Au belong to the same chemical group. More remarkably, Ag N with N ≥13 never formed at an unfaulted HUC, whereas Au 13 –Au 17 did form (see Fig. 4g–k ). When a diffusing Ag atom is transferred into a NS adjacent to Ag 12 as the arrow in Fig. 4b shows, it hops out quickly and diffuses among the three nearest neighbouring NSs surrounding Ag 12 (see Fig. 4c ). This suggests that the barrier associated with the single Ag atom diffusion to the nearest neighbouring NSs can be lowered by the presence of the Ag 12 cluster even without the tip’s close proximity effect (see Supplementary Fig. 3 , and Supplementary Notes 7 and 8 ). Although the route for these diffusions had to pass through the NS that held the Ag 12 cluster, Ag 13 never formed within the observable time scale. This is an indication that 12 is the maximum number of Ag atoms available for each NS of an unfaulted HUC. It is interesting to note that, when two Ag atoms are brought into a NS adjacent to Ag 12 , Ag 3 is formed instead of Ag 2 , as shown in Fig. 4d . The presence of the Ag 2 cluster in the nearby cell leads to a dissociation of one Ag atom from the Ag 12 , thereby producing two cluster arrays of Ag 11 and Ag 3 . The resulting Ag 3 diffuses in a concerted way among the three NSs surrounding the newly formed Ag 11 cluster. The appearance of the Ag 11 cluster accompanied by the formation of Ag 3 looks different from the isolated Ag 11 (compare Fig. 4a and Fig. 4d ; also see Supplementary Figs 3 and 4 , and Supplementary Notes 7 and 9 ). A preferential growth in the faulted HUC has been observed for the Au and Ag clusters formed by thermal annealing process in previous STM investigations [9] , [25] . On the contrary, with our gating method the clusters can be assembled equally on both the faulted and unfaulted HUCs, since the adsorbates are forcibly collected into a predetermined HUC. The fabrication method provided by the gating process can also be used to assemble multi-element clusters. The additional degree of freedom inherent in bimetallic clusters offers the opportunity to tune their structural and chemical properties by varying the cluster composition. The composition in the cluster can be designed and controlled atom-by-atom by identifying the atomic species adsorbed sequentially on surfaces from the SPM images. The bimetallic clusters involving metal atoms of two different species were assembled (see Supplementary Fig. 5 and Supplementary Note 10 ). An exemplary cluster of Au N Pb (with N =2–5) is displayed in Fig. 4l–o . The characteristic appearance of these mixed clusters departs considerably from their pure counterparts (see Fig. 2 and Supplementary Notes 6 and 11 ). The presence of the single Pb atom in Au 2 can stabilize the Au 2 Pb cluster, although Au 2 and Au 3 are mobile at RT. On the contrary, the Au 4 Pb and Au 5 Pb clusters exhibit two distinct features separated by partially stable round and fuzzy features in the STM images, whereas Au 4 –Au 6 are relatively stable (see Fig. 3a ). This result implies that a single Pb atom can stabilize a maximum of only two Au atoms in the NS. Accommodation of an additional number of Au atoms into this NS does not contribute to the clustering with Au 2 Pb, leaving the added Au atoms free to move. Thus, the Au 2 Pb cluster can be classified as a magic cluster due to its preference for staying intact without interaction with other Au atoms. These exemplary results clearly indicate that the stability of the clusters depends critically on the atomic species involved in the cluster structures. Valency of each component in a cluster dominates the bonding network and therefore determine the stability of the cluster. This fabrication technique can potentially be applied to the investigation of synergistic effects in bimetallic clusters [28] . It might be also possible to tune the reactivities of bimetallic clusters by varying the nature of the constituent atoms using the atom gating method, allowing the study of the reactivities of subnanoscale catalysis. We have demonstrated a new approach to the formation of various atom clusters with pre-designed composition at RT. The mechanism underlying this method was identified as a pure mechanical effect. The tip induces a reduction of the activation energy barrier between the adjacent NSs, allowing the diffusing atoms to jump into the desired NS, accompanied by atom trapping below the tip. This method provides access to investigate the dependence of a cluster’s stability on its size and composition. This technique, when combined with simultaneous AFM/STM characterization ability of submolecular level imaging [29] and of chemical identification [30] , may allow us to experimentally determine the structures of clusters. Atom gating is a highly controllable technique that can be applied to various adsorbates and surfaces possessing periodic NS arrays, such as graphene moiré pattern [31] , hexagonal boron nitride (h-BN) nanomesh [32] and alumina on Ni 3 Al(111) templates [33] . The cluster arrays formed on these templates are expected to have potential in both fundamental aspects and technological applications. These results serve as the basis for further investigations of the interplay between the sizes of supported clusters and their magnetic and catalytic properties. AFM/STM set-up and sample preparation The experiments were carried out with custom-built ultra-high-vacuum AFM/STM systems operated at RT [15] , [18] , equipped with versatile scan controllers [34] . Commercial Pt–Ir-coated Si cantilevers (NCLPt, NanoWorld) were used for static STM measurements (that is, without tip oscillation) and simultaneous AFM/STM measurements (that is, dynamic mode). For the particular case of AFM measurements, Si cantilevers without a metal coating were also used. Before use, the tip apex in both types of cantilevers was carefully cleaned by Ar ion sputtering. Cantilever deflection sensors are based on optical interferometers. For AFM measurements, we applied the frequency modulation detection method [35] , by which we detected Δ f of cantilevers oscillating at a constant amplitude. Bias voltage ( V s ) was applied to the sample with respect to the tip being held at virtual ground potential. The I t signal was measured from the tip. The experimental set-up is described in detail elsewhere [36] . Acquisition parameters are summarized in Supplementary Table . The Si(111)-(7 × 7) surface was prepared by a standard method of flashing and annealing. Various elements (Si, Sn, Pb, Ag and Au) were deposited onto the Si(111)-(7 × 7) surface by using a Joule heating evaporator in an ultra-high vacuum while the sample temperature was kept at RT (no further annealing process). Details of atom gating procedure The close proximity of the tip to the surface clearly affects atom transferring across the boundary. The success rate increases drastically with decreasing the tip–surface distance for atom gating process. A successful atom transferring by means of atom gating process takes place when the tip is approached towards the surface by about 3 Å from STM feedback position. We have empirically found that the location indicated by a cross in Fig. 1a is the most efficient site for transferring of the adsorbates presented in this study. On the other hand, the speed of vertical tip movement during the approach and retraction can also contribute to the probability of atom hopping between two NSs. The residence time of tip interaction with the target atom at the distance of closest approach to the surface increases by reducing the speed of vertical tip approach/retraction. Consequently, the rate of the atom hopping probability increases. How to cite this article: Sugimoto, Y. et al. Mechanical gate control for atom-by-atom cluster assembly with scanning probe microscopy. Nat. Commun. 5:4360 doi: 10.1038/ncomms5360 (2014).